Observation of a large spin-dependent transport length in organic spin valves at room temperature The integration of organic semiconductors and magnetism has been a fascinating topic for fundamental scientific research and future applications in electronics, because organic semiconductors are expected to possess a large spin-dependent transport length based on weak spin–orbit coupling and weak hyperfine interaction. However, to date, this length has typically been limited to several nanometres at room temperature, and a large length has only been observed at low temperatures. Here we report on a novel organic spin valve device using C 60 as the spacer layer. A magnetoresistance ratio of over 5% was observed at room temperature, which is one of the highest magnetoresistance ratios ever reported. Most importantly, a large spin-dependent transport length of approximately 110 nm was experimentally observed for the C 60 layer at room temperature. These results provide insights for further understanding spin transport in organic semiconductors and may strongly advance the development of spin-based organic devices. The manipulation and utilization of the spin polarization of electrons in organic semiconductors (OSs) has attracted considerable research interest for fundamental material science and potential applications. OSs are expected to possess a large spin-dependent transport (SDT) length due to their weak spin–orbit coupling and weak hyperfine interaction [1] , [2] , [3] , [4] , [5] , [6] . The SDT phenomenon at room temperature via a tunnelling mechanism has been studied in several different OSs [7] , [8] , [9] , [10] , [11] , [12] . Nevertheless, the thickness of the OS layer is generally limited to around several nanometres, as the magnetoresistance (MR) ratio decays sharply, and subsequently disappears with increasing OS thickness. The observation of SDT in OSs in the hopping process has also been reported [2] , [3] in such materials as tris(8-hydroxyquinolinato) aluminium (Alq 3 ) and rubrene. However, most studies have only been carried out at low temperatures because of the evident reduction in the SDT length with increasing measurement temperatures until the MR effect finally disappears at room temperature [2] , [13] , [14] , [15] , [16] , [17] , [18] , [19] . Thus, whether a large SDT length can be realized in OSs at room temperature remains unclear. The traditional optical pump–probe method used for studying spin dynamics and transport in inorganic semiconductors is not suitable for OSs because of the weak spin–orbit interaction and the absence of a crystalline structure with inversion asymmetry in OSs [16] , [17] . The use of an organic spin valve device is still the most popular technique for investigating SDT in OSs [2] . An organic spin valve is a multilayer device composed of two ferromagnetic (FM) electrodes separated by an OS spacer layer. The spin valve exhibits the MR phenomenon, that is, the change in electrical resistance depends on the magnetization alignment of the two FM electrodes. Thus, the device can be used to directly investigate the SDT properties of OSs by measuring the MR effect. Here we report on a novel organic spin valve device with an MgO substrate/Fe 3 O 4 /Al-O/C 60 /Co/Al stacking structure; we studied spin injection, transport and detection in the device. An MR ratio greater than 5% was observed at room temperature, which is one of the highest MR ratios reported to date [7] , [8] , [10] , [11] , [12] , [13] . Most importantly, a large SDT length of approximately 110 nm was experimentally observed in the C 60 layer at room temperature. This research may strongly motivate the development of spin-based organic devices, such as organic spin valves [1] , [2] , [3] , [4] , [5] , [6] , [7] , [8] , [9] , [10] , [11] , [12] , [13] , [14] , [15] and spin-based organic light-emitting diodes [20] . Device structure Here we report on a functional organic spin valve device with an MgO substrate/Fe 3 O 4 /Al-O/C 60 /Co/Al stacking structure. A schematic diagram of the spin valve structure that was investigated is shown in Fig. 1a . Fe 3 O 4 was selected as the bottom FM electrode, because density-functional calculations show that the electrons of Fe 3 O 4 at the Fermi level are 100% spin-polarized [21] , [22] , which is suitable for efficient spin injection even though the actual spin polarization of Fe 3 O 4 is affected by the contact interface [23] , [24] , [25] , [26] , [27] . The Verwey transition temperature was observed to be 117 K for a Fe 3 O 4 film ( Supplementary Fig. S1 ), confirming the high quality of the film. A stable Al-O layer was used to protect the surface of the Fe 3 O 4 layer for mask exchange and increased spin injection efficiency. A C 60 molecule was used as the organic layer, and Co was used as the top FM electrode. C 60 is stable and easily forms a high-quality molecular film via thermal evaporation. In particular, the hyperfine interaction in C 60 is considerably weak because of the absence of polarized hydrogen nuclei and the low natural abundance of 13 C nuclear spins in the C 60 molecule [11] , [12] , [14] , [15] . The weak hyperfine interaction has been predicted to increase the SDT length [28] , which has been demonstrated at low temperatures using a deuterated polymer as a spacer in organic spin valve devices [29] . In addition, the C 60 molecule is nearly isotropic because of its high symmetry and rotational freedom. Therefore, a polarized electron can easily move from one molecule to the next with a smaller spin flip, because the energy loss of the carrier is small between hopping states [30] compared with other strongly anisotropic OSs, such as Alq 3 . These characteristics of C 60 can potentially increase the SDT length in spin-based organic devices. Furthermore, the energy levels of Fe 3 O 4 , C 60 and Co are well matched, as shown in Fig. 1b . Thus, in principle, electron spin injection, transport and detection can be realized in the present organic spin valve device. 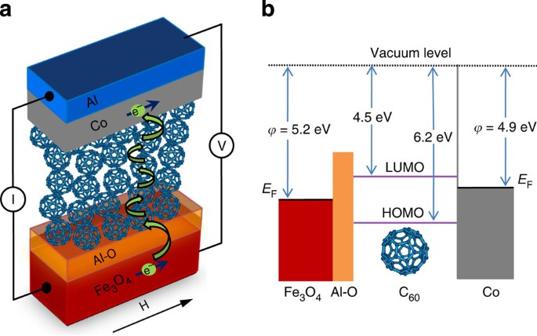Figure 1: Structure of designed organic spin valve devices. (a) Schematic diagram of the device structure with an MgO substrate/Fe3O4/Al-O/C60/Co/Al stacking structure. (b) Schematic band diagram of the organic device in the rigid band approximation shows the Fermi levels (EF), the work functions of the two ferromagnetic electrodes (Fe3O4and Co), the highest occupied molecular orbital (HOMO) and the lowest unoccupied molecular orbital (LUMO) levels of C60. Figure 1: Structure of designed organic spin valve devices. ( a ) Schematic diagram of the device structure with an MgO substrate/Fe 3 O 4 /Al-O/C 60 /Co/Al stacking structure. ( b ) Schematic band diagram of the organic device in the rigid band approximation shows the Fermi levels ( E F ), the work functions of the two ferromagnetic electrodes (Fe 3 O 4 and Co), the highest occupied molecular orbital (HOMO) and the lowest unoccupied molecular orbital (LUMO) levels of C 60 . 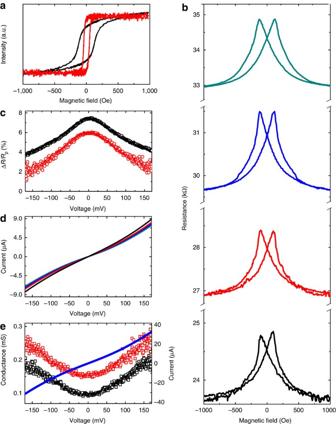Figure 2: Hysteresis curves and transport properties of organic spin valve devices. (a) Hysteresis curves for individual electrodes Fe3O4(black curve) and Co (red curve), which were measured at 300 K. (b) Magnetoresistance curves of the organic device composed of a 80-nm-thick C60layer measured at different temperatures, showing magnetoresistance ratios of 5.3% at 300 K (black curve), 6.1% at 250 K (red curve), 6.7% at 200 K (blue curve) and 6.9% at 150 K (dark cyan curve). The bias voltage was fixed at 30 mV to measure the magnetoresistance effect. (c) Bias-voltage dependence of ΔR/Rpat 300 K (red circles) and 150 K (black circles) for a device with of a 80-nm-thick C60layer. (d) Nonlinear current–voltage curves for the device with a 80-nm-thick C60layer at 300 K (black curve), 250 K (red curve), 200 K (blue curve) and 150 K (dark cyan curve). (e) Conductance versus bias curves for a device with a 10-nm-thick C60layer measured at 300 K (red squares) and 150 K (black squares), and the corresponding nonlinear current–voltage curve (blue circles) at 300 K. Full size image Hysteresis curves and spin transport properties Figure 2a shows the hysteresis curves for the individual electrodes of Fe 3 O 4 and Co, which were measured at 300 K. Coercivities near 140 and 40 Oe for Fe 3 O 4 and Co, respectively, can be clearly observed. The different coercivities induce magnetization alignments with antiparallel and parallel alignments in the organic spin-valve devices ( Supplementary Fig. S2 ), providing a precondition for investigating the MR effect. The MR curves for the device with an 80-nm-thick C 60 layer measured at 300, 250, 200 and 150 K are shown in Fig. 2b . As expected, at 300 K, MR peaks appeared at around ±100 Oe, in good agreement with the observations in Fig. 2a and Supplementary Fig. S2 . The MR gradually decreased on either side towards the large-field value ( Fig. 2b ). In spin-valve devices, the shape of the MR curve depends on the angle θ between the magnetization moments of two FM electrodes [31] , [32] , [33] . If the hysteresis curves of both electrodes have ideally rectangular shapes, θ can take only two values, 0° and 180°. In general, a smaller and larger MR appear when the magnetization alignment is parallel ( θ is 0°) and antiparallel ( θ is 180°), respectively. In contrast, if the hysteresis curves of electrodes are not ideally rectangular, particularly for Fe 3 O 4 , θ will take other values (0°< θ <180°), as shown in Fig. 2a . In this case, the MR is continuously reduced with decreasing θ until θ equals 0° ( Fig. 2b ). Figure 2: Hysteresis curves and transport properties of organic spin valve devices. ( a ) Hysteresis curves for individual electrodes Fe 3 O 4 (black curve) and Co (red curve), which were measured at 300 K. ( b ) Magnetoresistance curves of the organic device composed of a 80-nm-thick C 60 layer measured at different temperatures, showing magnetoresistance ratios of 5.3% at 300 K (black curve), 6.1% at 250 K (red curve), 6.7% at 200 K (blue curve) and 6.9% at 150 K (dark cyan curve). The bias voltage was fixed at 30 mV to measure the magnetoresistance effect. ( c ) Bias-voltage dependence of Δ R/R p at 300 K (red circles) and 150 K (black circles) for a device with of a 80-nm-thick C 60 layer. ( d ) Nonlinear current–voltage curves for the device with a 80-nm-thick C 60 layer at 300 K (black curve), 250 K (red curve), 200 K (blue curve) and 150 K (dark cyan curve). ( e ) Conductance versus bias curves for a device with a 10-nm-thick C 60 layer measured at 300 K (red squares) and 150 K (black squares), and the corresponding nonlinear current–voltage curve (blue circles) at 300 K. Full size image The MR ratio was calculated using the expression Δ R/R p =( R ap /R p −1) × 100%, where R ap and R p denote the resistance in the antiparallel and parallel states, respectively. The R p value was obtained at a magnetic field of 3,000 Oe. The calculation shows an MR ratio of 5.3% at 300 K, which is one of the highest MR ratios that have been reported at room temperature [7] , [8] , [10] , [11] , [12] , [13] . Note that both the MR ratios and device resistance increased with decreasing measurement temperatures. The MR ratios were 6.1% at 250 K, 6.7% at 200 K and 6.9% at 150 K. The bias-voltage dependence of the MR ratio at 300 and 150 K is shown in Fig. 2c . The clearly nonlinear nature of the current–voltage curves can be observed in Fig. 2d . Similar conductance-bias curves were observed at 300 and 150 K for the device with a 10-nm-thick C 60 layer, as shown in Fig. 2e . The primary difference was the downshift of the curve at 150 K due to the increase in the resistance, indicating that the C 60 layer may have been free of magnetic inclusions [7] . A detailed analysis about the nonlinear behaviors of current-voltage curves in Fig. 2d and 2e can be found in the Supplementary Discussion . Microstructure of an organic device To further explore the microstructure of the organic spin-valve devices, scanning transmission electron microscopy and elementary mapping by energy dispersive X-ray spectroscopy were performed for an organic spin-valve device. The microscopy images of Fig. 3a show that each layer had a sharp interface and that the C 60 layer was homogeneous. The elementary mappings of C, Co and Al showed a clear separation for each layer, as shown in Fig. 3b–d , respectively. These studies further demonstrate that there was no appreciable diffusion of Co into the C 60 layer. Thus, it is very likely that the ‘ill-defined’ layer due to metal inclusions that is assumed for the organic layer in Alq 3 -based spin valve devices [2] does not appear in our devices. One possible reason for the absence of this layer is the difference between the spatial structures of the C 60 and Alq 3 molecules ( Supplementary Fig. S3 ). The spherical structure of C 60 makes the sustenance of the upper metallic layer easy. The ‘ill-defined’ layer may also be related to the fabrication methods [7] , [8] , [10] , [29] . The Raman spectrum for the C 60 layer was measured for an organic spin valve device ( Supplementary Fig. S4 ), confirming the typical molecular characteristics of C 60 . 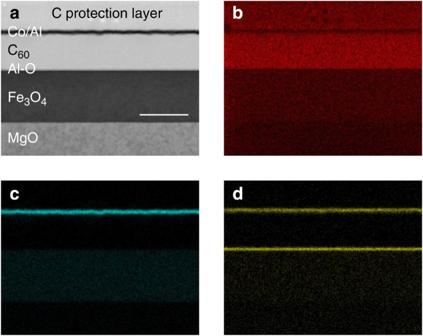Figure 3: Microstructure of an organic spin valve device. (a) Scanning transmission electron microscopy of a device with an MgO substrate/Fe3O4/Al-O/C60/Co/Al stacking structure; the top C layer was deposited to protect the device layers during microscopy measurements. Scale bar, 100 nm. Panelsb–dare the elementary mappings of C (red), Co (cyan) and Al (yellow), respectively, for K-shell electrons performed by energy dispersive X-ray spectroscopy. Figure 3: Microstructure of an organic spin valve device. ( a ) Scanning transmission electron microscopy of a device with an MgO substrate/Fe 3 O 4 /Al-O/C 60 /Co/Al stacking structure; the top C layer was deposited to protect the device layers during microscopy measurements. Scale bar, 100 nm. Panels b – d are the elementary mappings of C (red), Co (cyan) and Al (yellow), respectively, for K-shell electrons performed by energy dispersive X-ray spectroscopy. Full size image Demonstration of MR effect originates from spin valve device The MR effect could also arise from the anisotropic MR effects of the FM electrodes themselves. Therefore, the anisotropic MR ratios for the full length of the Fe 3 O 4 and Co strips were evaluated. The anisotropic MR ratios were found to be approximately −0.04 and 0.12% for the Fe 3 O 4 and Co layers, respectively ( Supplementary Fig. S5 ). These values were 40 times lower than the MR ratios of the organic spin valve devices, which demonstrates that the observed MR ratio was not due to the anisotropic MR effect. Meanwhile, a spin valve-like MR phenomenon, known as tunnelling anisotropic MR [34] , was examined by fabricating the devices with an MgO substrate/Fe 3 O 4 /Al-O/C 60 /Al stacking structure. There were no tunnelling anisotropic MR effects in these devices ( Supplementary Fig. S6 ). On the basis of this systemic investigation, the MR effect in our organic spin valve devices could conclusively be attributed to the SDT of the C 60 layer. Dependence of MR ratio on C 60 thickness A set of organic spin valve devices consisting of different C 60 layer thicknesses (10–110 nm) were fabricated. The measured MR curves were similar to that shown in Fig. 2b for all devices ( Supplementary Fig. S7 shows one such curve). The dependence of the MR ratio on the C 60 layer thickness at 300 and 150 K is plotted in Fig. 4a . The MR ratios at 150 K were larger than those at 300 K for each corresponding C 60 layer thickness due to the decrease in spin scattering (such as magneto-excitation) at lower temperatures. Notably, an unusual and interesting dependence of the MR ratio on the C 60 layer thickness was observed, which differs from previous reports. The MR ratios sharply increased upon increasing the C 60 layer thickness from 10 to 40 nm and then slowly increased for increases in the C 60 layer up to 80 nm. Beyond this range, further increases in the C 60 layer thickness produced a drastic reduction in the MR ratio. Fortunately, a C 60 layer thickness of 110 nm was successfully observed with an MR ratio of approximately 0.5% at room temperature in the devices. To the best of our knowledge, this thickness is the largest SDT length reported at room temperature in OSs with vertical spin valve structures to date. We suggest that when compared with other reported OSs, such as rubrene and Alq 3 , the weaker spin–orbit coupling and hyperfine interaction of the C 60 molecule [14] , [28] , [29] significantly reduces spin flip in the organic film. Thus, a large SDT length was obtained for the C 60 layer. Our results indicate that the SDT length relies strongly on the molecular configuration of the OS. 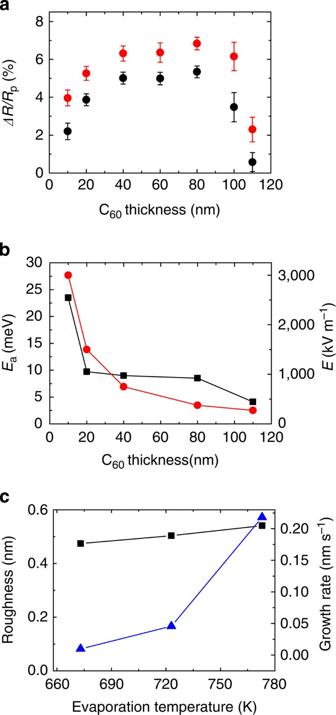Figure 4: Thickness and temperature dependence. (a) ΔR/Rpas a function of the C60layer thickness measured at 300 K (black circles) and 150 K (red circles). The bias voltage was fixed at 30 mV to measure magnetoresistance effect. Error bar represent one standard deviation of ΔR/Rpfor every thickness and is estimated based on the scatter in the date of ΔR/Rpfrom four devices at each thickness. (b) Activation energy (black squares) and electric field magnitude (red circles) as a function of the C60layer thickness. (c) Dependence of the roughness (black squares) and growth rate (blue triangles) on the evaporation temperature for the 80-nm-thick C60films; the solid curves inbandcare only visual guides. Figure 4: Thickness and temperature dependence. ( a ) Δ R/R p as a function of the C 60 layer thickness measured at 300 K (black circles) and 150 K (red circles). The bias voltage was fixed at 30 mV to measure magnetoresistance effect. Error bar represent one standard deviation of Δ R/R p for every thickness and is estimated based on the scatter in the date of Δ R/R p from four devices at each thickness. ( b ) Activation energy (black squares) and electric field magnitude (red circles) as a function of the C 60 layer thickness. ( c ) Dependence of the roughness (black squares) and growth rate (blue triangles) on the evaporation temperature for the 80-nm-thick C 60 films; the solid curves in b and c are only visual guides. Full size image To analyse the dependence of the MR ratio on the C 60 layer thickness, the structures of the C 60 layers were studied. X-ray diffraction measurements showed that the C 60 layers of different thickness were structurally amorphous. The C 60 layer thickness in our devices was far greater than the tunnelling barrier limit that has been reported thus far [7] , [8] , [9] , [10] , [11] , [12] , [35] . Thus, the SDT within the C 60 layer via hopping between localized neighbouring states was mainly considered. Our results can therefore be described by the Gaussian disorder model. Bobbert et al. [28] presented a theory for spin transport in disordered OSs. The authors concluded that both the spin diffusion length ( l s ) and mobility ( μ ) decreased with a decreasing electric field ( E ) ( E <5[σ/ea]). E was determined by the equation E = U / d , where U and d are the applied voltage and distance between two electrodes, respectively. In our spin valve devices, U was fixed at 30 mV and d was determined by the C 60 layer thickness. Thus, as the C 60 layer thickness increased, E decreased, as shown in Fig. 4b . As a result, l s and μ decreased. Bobbert et al. [28] also suggested that l s and μ increase with decreasing disorder strength. The activation energy ( E a ) is a direct reflection of the amount of disorder strength [36] . The E a of C 60 was estimated from the temperature dependence of the resistance ( Supplementary Fig. S8 ) and is plotted in Fig. 4b . E a clearly decreased with increasing C 60 thickness, indicating that the disorder strength of the C 60 layer decreased. This result indicates that l s and μ increased with increasing C 60 thickness. The competition between these two factors ( E and disorder) likely leads to a maximum for both l s and μ . As l s and μ increase, the dependence of MR on the magnetization alignments of the two electrodes becomes stronger, which is the origin of the MR effect [28] . Consequently, a maximum of ΔR/R p can appear with increasing C 60 layer thickness. The change ratios for l s and μ were distinctly different for different values of E (ref. 28 ). This observation could explain the different increasing slopes of ΔR/R p for C 60 layer thicknesses of 10–40 nm and 40–80 nm. The decrease in E a implies that the molecular interactions between C 60 molecules may vary. In our organic spin valve devices, E a was smaller than the values reported in the literature [37] , likely because of the dependence of the mobility on the charge-carrier density induced by different devices [36] , [37] . To estimate l s in the organic spin valve devices, the MR signals were tentatively fitted by the following formula [28] , [29] , MR( B )=0.5 × MR max [1− m 1 ( B 1 ) × m 2 ( B 2 )]exp(− d / l s ), where MR max is the MR when spin relaxation is neglected, d is the thickness of the organic spacer, m 1 ( B 1 ) and m 2 ( B 2 ) denote the normalized magnetizations of the FM electrodes, l s = l s,0 × [1+( B/B 0 ) 2 ] 3/8 , B is the applied magnetic field and B 0 is a characteristic field related to hyperfine interaction. One fit for a device with d =80 nm at 300 K and 30 mV is shown in Supplementary Fig. S9 . It produces that l s,0 / d is ~1.7 and MR max is ~9%. The maximum MR ratio appears for B at ±100 Oe. Thus, the fit predicts that the largest l s value is approximately 150 nm at room temperature in our devices. On the basis of the fit values for MR max and l s , the MR was calculated using MR=MR max × exp(− d / l s ). As shown in Supplementary Fig. S10 , the dependence of the calculated MR ratio on the C 60 layer thickness basically agrees with our experiments. It should be pointed out that these estimated values likely include a fitting error, because the fitting is not very exact ( Supplementary Fig. S9 ). The above fitting formula results from the random hyperfine coupling and Zeeman coupling [28] . Thus, one possible reason for the presence of fitting error is that other interactions, such as the exchange interaction or/and spin–orbit coupling, also contribute to the spin transport in OSs, as was suggested in [29] and studied in [38] . Further studies are needed to clarify the effect of these other interactions on spin transport in detail. The interfaces between the FM electrodes and molecular layer determine the spin injection and detection efficiency, and thus significantly affect the MR ratio of organic spin valve devices. Spin valve devices with an MgO substrate/Fe 3 O 4 /C 60 /Co/Al stacking structure (without an Al-O layer) were fabricated. However, the MR effect did not appear in these devices ( Supplementary Fig. S11 ), likely because of the decrease in the spin polarization of Fe 3 O 4 resulting from surface degradation ( Supplementary Fig. S12 ). The thin Al-O film is very stable in air and has been known as an efficient barrier [33] , [39] . Inserting an Al-O layer to protect the Fe 3 O 4 produced the MR effect in our spin valve devices. With the same device size, the spin valve with an Al-O layer but lacking a C 60 layer also did not show an MR effect originating from the device ( Supplementary Fig. S5 ). The evaporation temperature of the C 60 layers was 723 K for the organic spin valve devices reported above. We found that the evaporation temperature of the C 60 layer had an essential role in modifying the SDT properties. Organic spin valve devices with an 80-nm-thick C 60 layer were also fabricated by evaporating C 60 at 673 and 773 K. Both series of devices showed MR ratios of approximately 1.7% at room temperature. These MR ratios were three times smaller than that of the device with C 60 evaporated at 723 K. Note that the R p of the devices with C 60 evaporated at 673 K was approximately 12.5 kΩ, which was approximately two times smaller than that of the devices with C 60 evaporated at 723 K. In contrast, the R p of the device with C 60 evaporated at 773 K was nearly 1 MΩ. The resistance was inversely proportional to the carrier mobility. The decrease of R p at 673 K did not lead to an increase in the MR ratio, indicating that the MR ratio was not solely affected by the carrier mobility, in agreement with the analysis for Fig. 4a , as well as the literature [38] . The roughness and growth rates of the C 60 films for different evaporation temperatures are plotted in Fig. 4c . The roughness for all films was approximately 0.5 nm, which is less than the diameter of a C 60 molecule (approximately 1 nm), indicating that the films were extremely smooth. However, the growth rates were significantly different, corresponding to 0.015, 0.045 and 0.22 nm s −1 for the films evaporated at 673, 723 and 773 K, respectively. These differences can be attributed to the different kinetic energies for the C 60 molecules obtained at each evaporation temperature. The kinetic energy of the molecules clearly affected the thermal equilibrium of the individual C 60 molecules when the final film formed. Thus, the molecular distance and intermolecular interactions in organic films will vary for different temperatures. The intermolecular distance and interactions may affect the orbital overlap of the π electrons in OSs [40] , which determine the transport efficiency of the charge carriers. Previous studies have also reported that temperature affects the lattice fluctuations [41] , [42] and intramolecular interactions [30] , [43] of C 60 , which may cause variations in the σ -orbital. The σ -orbital affects the SDT length in organic OSs [38] . Moreover, the C 60 molecule exhibits a series of energy levels [41] . The evaporation temperature may affect the distribution of the energy levels in a C 60 layer. This energy redistribution can reduce the matching of energy levels between the C 60 molecules for hopping transport, thus decreasing the hopping efficiency of the C 60 layer. Meanwhile, the energy redistribution may also change the interactions between the C 60 energy levels and electrodes at the interfaces, leading to lower spin injection and/or detection efficiencies. This study has shown that the microstructure in organic spin valve devices is closely correlated with magnetotransport, in agreement with the literature [44] . On the basis of an optimized evaporation temperature for the C 60 layer at 723 K, we deduced that an efficient SDT pathway exists in a spin valve device with a C 60 layer of 80 nm for achieving a high MR ratio in which spin electrons are efficiently injected [17] , [45] into the C 60 layer and hopping transport occurs with very a small spin flip, as illustrated in Fig. 5 . The most recent theoretical investigation predicts that an SDT length of more than 430 nm for C 60 can be achieved at room temperature [46] . Our results are consistent with this theoretical study. In the organic spin valve devices considered here, the C 60 layer had an amorphous structure. Thus, a larger SDT length for C 60 layers at room temperature can be expected when C 60 forms a single crystalline structure. 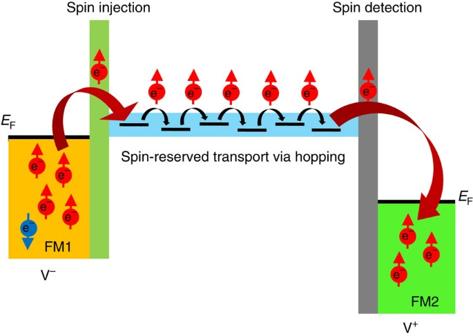Figure 5: Illustration of an efficient spin-reserved transport pathway. Excellent matching of energy levels within the C60layer for spin-reserved transport via a hopping mechanism, and the interfaces between the FM electrodes and C60layer result in high efficiencies for spin injection/detection under optimized fabrication conditions. Figure 5: Illustration of an efficient spin-reserved transport pathway. Excellent matching of energy levels within the C 60 layer for spin-reserved transport via a hopping mechanism, and the interfaces between the FM electrodes and C 60 layer result in high efficiencies for spin injection/detection under optimized fabrication conditions. Full size image In conclusion, we have shown that a large SDT length of approximately 110 nm for C 60 can be realized in room-temperature experiments. The large SDT length is likely governed by the weak hyperfine interactions of the C 60 molecule. The spin injection/detection efficiency at the interface of the electrode/molecule together with the molecular interactions determines the value of the MR ratio. Such an investigation furthers our understanding of spin transport in OSs and could be pivotal in the development of spin-based molecular electronics for future applications. Sample fabrication The Fe 3 O 4 (70 nm) electrode was deposited using ultrahigh-vacuum magnetron sputtering (at a base pressure of 10 −9 Torr) with a shadow mask to form a strip on an MgO (001) substrate. Al (2 nm) was deposited on the MgO substrate/Fe 3 O 4 layer in the same chamber, followed by immediate oxidization by exposure to oxygen plasma to obtain an Al-O layer. The MgO substrate/Fe 3 O 4 /Al-O film was removed from the chamber, and then the mask was removed in air. The film was then installed into the thermal evaporation chamber (base pressure <10 −6 Torr) for molecular deposition. A new shadow mask was used to form a rotund C 60 layer (99.9%, Strem Chemicals Inc.). The MgO substrate/Fe 3 O 4 /Al-O/C 60 layers were transferred to a different chamber, without breaking the vacuum, to deposit a Co layer (10 nm) via magnetron sputtering (base pressure <10 −7 Torr; Ar ion plasma). A third shadow mask was inserted to form a Co strip for patterning a cross configuration. Finally, Al (5 nm) was deposited to prevent oxidation of the Co layer. The top Co/Al layer was deposited at a very low electric power (10 W) to reduce the kinetic energy of the Co and Al atoms. The substrate was rotated using a mechanical motor during the deposition for each layer to homogenize the film. The fabricated device area was 1.5 × 1.5 mm 2 . Experimental setup Transport properties were measured via the standard four-probe method using a physical property measurement system (Quantum Design). The crystal structures for the thin films were characterized using X-ray diffraction (Smartlab, Rigaku Co.). The magnetization curves were measured using a vibrating-sample magnetometer with an applied field parallel to the film plane. The film roughness was characterized by atomic force microscopy (SII Seiko Instruments, SPA 400). Scanning transmission electron microscopy was performed using a HD-2700 (Hitachi Co.) with the acceleration voltage set at 200 kV. Elementary mapping was performed by energy dispersive X-ray spectroscopy (HD-2700) with the accelerating voltage set at 200 kV and an Si/Li detector. Raman spectroscopy was performed using a LabRAM HR 800 Raman Spectrometer (Horiba Jobin Yvon Co.) with the Ar + laser wavelength set at 514.5 nm. How to cite this article: Zhang, X. et al. Observation of a large spin-dependent transport length in organic spin valves at room temperature. Nat. Commun. 4:1392 doi: 10.1038/ncomms2423 (2013).